Rudimentary substrates for vocal learning in a suboscine Vocal learning has evolved in only a few groups of mammals and birds. The key neuroanatomical and behavioural links bridging vocal learners and non-learners are still unknown. Here we show that a non-vocal-learning suboscine, the eastern phoebe, expresses neural and behavioural substrates that are associated with vocal learning in closely related oscine songbirds. In phoebes, a specialized forebrain region in the intermediate arcopallium seems homologous to the oscine song nucleus RA (robust nucleus of arcopallium) by its neural connections, expression of glutamate receptors and singing-dependent immediate-early gene expression. Lesion of this RA-like region induces subtle but consistent song changes. Moreover, the unlearned phoebe song unexpectedly develops through a protracted ontogeny. These features provide the first evidence of forebrain vocal-motor control in suboscines, which has not been encountered in other avian non-vocal-learners, and offer a potential configuration of brain and behaviour from which vocal learning might have evolved. Vocal learning has evolved in only three clades of birds, the oscine songbirds (order Passeriformes), parrots (Psittaciformes) and hummingbirds (Apodiformes) [1] , [2] ( Fig. 1a ). The origin and evolution of this complex learned behaviour remains unclear. Vocal learning is characterized by its dependence on intact hearing [3] , a protracted vocal ontogeny [4] , and a specialized forebrain circuitry [5] that innervates vocal and respiratory nuclei of the brainstem and presides over the acquisition and production of learned song ( Fig. 1b ). These behavioural and neuroanatomical traits have not been found in non-vocal-learners [6] , which develop species-specific vocalizations in the absence of hearing [7] , and have no known forebrain vocal-motor control [8] , [9] . In non-vocal-learners, the vocal pathway is thought to consist solely of midbrain and brainstem nuclei [9] , [10] , [11] . One of the neuroanatomical missing links for vocal learning to occur is thus the lack of projections from the telencephalon directly to vocal/respiratory neurons in the brainstem [12] , [13] . In non-vocal-learners, the forebrain nucleus Ai (intermediate arcopallium) has been considered most comparable to song nucleus RA (robust nucleus of arcopallium) in oscines, as Ai has motor-related projections to midbrain/hindbrain [14] . However, studies from several groups of non-learning birds show that Ai does not project to brainstem vocal and respiratory nuclei [15] , [16] . 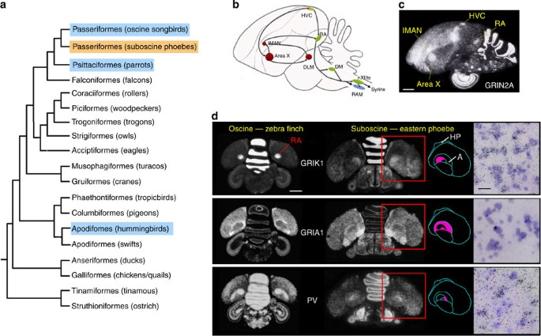Figure 1: Specialized gene expression in the forebrain region of a suboscine bird is similar to vocal learners. (a) Avian phylogeny according to DNA sequences of 19 nuclear loci; the three clades of vocal learners are highlighted in blue54. The suboscines of Passeriformes (light orange) are the closest relatives of oscines and most of them are non-vocal-learners. (b) Schematic representation of the song system of oscines in sagittal view. The song system consists of the anterior forebrain circuit (red) and the vocal-motor pathway (green), both diverge from nucleus HVC. The vocal-motor pathway projects to a respiratory nucleus RAm in the brainstem (blue). (c) Example of differential expression of a glutamate receptor subunit (GRIN2A) in the four major forebrain song nuclei shown here for an oscine, the chipping sparrow (sagittal view). (d) Inverted autoradiograph images ofin situhybridization comparing the mRNA expression pattern (white label) in coronal sections of the arcopallium of a zebra finch and eastern phoebe male. The RA-like specialization and an adjacent portion of the Ai of the phoebes are highlighted in the drawings to the right. Note the increased expression ofGRIK1andPVin the zebra finch RA nucleus, and increased expression ofGRIK1in the phoebe RA-like region. Scale bar,1 mm. The right panel shows higher magnification of the RA-like region in phoebes showing the presence of silver grains, counterstained with cresyl violet Nissl staining (purple). The neurons in RA-like region are bigger than the surrounding cells. Scale bar, 200 μm. Anatomical abbreviations: DLM, nucleus dorsolateralis anterior thalamis; LMAN, lateral magnocellular nucleus of the anterior nidopallium; nXIIts, tracheosyringeal hypoglossal nucleus. Scale bar, 1 mm. Figure 1: Specialized gene expression in the forebrain region of a suboscine bird is similar to vocal learners. ( a ) Avian phylogeny according to DNA sequences of 19 nuclear loci; the three clades of vocal learners are highlighted in blue [54] . The suboscines of Passeriformes (light orange) are the closest relatives of oscines and most of them are non-vocal-learners. ( b ) Schematic representation of the song system of oscines in sagittal view. The song system consists of the anterior forebrain circuit (red) and the vocal-motor pathway (green), both diverge from nucleus HVC. The vocal-motor pathway projects to a respiratory nucleus RAm in the brainstem (blue). ( c ) Example of differential expression of a glutamate receptor subunit ( GRIN2A ) in the four major forebrain song nuclei shown here for an oscine, the chipping sparrow (sagittal view). ( d ) Inverted autoradiograph images of in situ hybridization comparing the mRNA expression pattern (white label) in coronal sections of the arcopallium of a zebra finch and eastern phoebe male. The RA-like specialization and an adjacent portion of the Ai of the phoebes are highlighted in the drawings to the right. Note the increased expression of GRIK1 and PV in the zebra finch RA nucleus, and increased expression of GRIK1 in the phoebe RA-like region. Scale bar,1 mm. The right panel shows higher magnification of the RA-like region in phoebes showing the presence of silver grains, counterstained with cresyl violet Nissl staining (purple). The neurons in RA-like region are bigger than the surrounding cells. Scale bar, 200 μm. Anatomical abbreviations: DLM, nucleus dorsolateralis anterior thalamis; LMAN, lateral magnocellular nucleus of the anterior nidopallium; nXIIts, tracheosyringeal hypoglossal nucleus. Scale bar, 1 mm. Full size image The evolutionary origin of complex behavioural traits, such as vocal learning, can be better understood through examination of homologous neural circuits shared by closely related species [17] . To bridge the neuroanatomical link between vocal learners and non-learners, we studied two closely related Passeriformes subgroups: the vocal-learning oscines and non-learning suboscines ( Fig. 1a ). While all oscines are thought to have vocal learning, most suboscines are thought to lack this learning plasticity and lack the discrete forebrain nuclei that are associated with vocal learning in oscines [18] , [19] , [20] , [21] . However, at least a few suboscine species, such as the three-wattled bellbird ( Procnias tricarunculata, of Cotingidae) and the long-tailed manakin ( Chiroxiphia linearis , of Pipridae), show vocal matching or song geographic variation [22] , [23] , [24] , suggesting that vocal learning may have evolved in these groups as well, but the underlying neural substrates remain unknown. In this study, we chose a suboscine, the eastern phoebe ( Sayornis phoebe) , to look for the antecedents of vocal learning. Previous studies have shown that the phoebe does not learn its song and can develop a species-specific song in the absence of hearing [18] , [25] , [26] . Here, we closely examine the neural circuits and song behaviours in the suboscine phoebes. We provide the first evidence that non-vocal-learning phoebes possess some of the forebrain vocal/respiratory control that are required for vocal learning in oscines. In addition, phoebes produce an unexpected, protracted period of plastic song before song crystallization. These behavioural and neural substrates of suboscine phoebes have not been identified in other non-vocal-learners and may represent rudimentary traits of vocal-learning songbirds. Expression of glutamate receptor genes in RA-like region First, we tested for differential messenger RNA expression of glutamate receptor subunits in the forebrain of phoebes. Glutamate receptors are necessary for glutamate-mediated excitation of neural cells and have a major function in the modulation of synaptic plasticity, which has strong implications for learning and memory [27] . Four subunits, GRIA1 , GRIK1 , GRM2 and GRIN2A (previously known as GluR1 , GluR5 , mGluR2 and NR2A ), were chosen for this study because they represent each of four glutamate receptor families (α-amino-3-hydroxy-5-methyl-4-isoxazolepropionic acid receptor (AMPA), kainite, metabotropic and N -methyl- D -aspartate), and they are differentially expressed in the forebrain song nuclei of the oscine’s song system [28] . We found the expression pattern of GRIK1 revealed a specialized RA-like region of the ventromedial Ai of phoebes ( n =3 males, 2 females; Fig. 1d and Supplementary Fig. S1 ), consisting of increased GRIK1 expression relative to the surrounding arcopallium, similar to that of the RA of oscines. However, the expression was more diffuse than in the RA of songbirds, in which a sharp cutoff in expression coincides with an easily recognizable cytoarchitectonic boundary of the song nucleus. As with the RA of songbirds, GRIA1 had decreased expression in the RA-like area and also in the Ai laterally adjacent to ‘RA’ ( Fig. 1d ). Two other subunits, GRM2 and GRIN2A , were widely expressed over most of the arcopallium in phoebes as in songbirds, and revealed no specialized RA-like area ( Supplementary Fig. S1 ). In addition, none of these subunits consistently identified potential homologues for the other major forebrain song nuclei in songbirds (such as high vocal center (HVC) and Area X). In two other non-vocal-learning birds, the Gambel’s quail, Callipepla gambelii (order Galliformes) and previously reported ringdoves [28] , Streptopelia risoria (order Columbiformes), expression of these glutamate receptor genes did not reveal any narrowly defined region in the arcopallium ( Supplementary Fig. S1 ). We also examined the expression of parvalbumin ( PV ), a calcium-binding protein, that is expressed in the nucleus RA analogues of all three vocal-learning clades [29] , [30] . In phoebes, we did not find differential PV expression in the GRIK1 -rich region of the arcopallium, but PV had higher expression in the lateral part of Ai as in songbirds ( Fig. 1d ). Singing induces immediate early genes expression in the RA-like region The GRIK1 -rich RA-like region of the phoebe arcopallium is associated with singing. Neural activity-regulated immediate early genes (IEGs), Arc and Egr1 , were examined under three experimental conditions: (1) singing and hearing song; (2) hearing song only; and (3) silent controls. Arc is an activity-regulated cytoskeletal-associated protein that acts at recently activated synapses and is involved in the synaptic plasticity of long-term potentiation in mammals [31] , [32] . In oscines, Arc is upregulated in the nucleus RA by singing, but not hearing of song or under silent conditions [33] . In singing phoebes ( n =4 birds), Arc showed significantly higher expression in the GRIK1 -rich RA-like region, compared to silent or song-hearing phoebes ( n =3 birds per group; one-way analysis of variance (ANOVA); P <0.01; Fig. 2 ). The amount of singing was positively correlated with the level of Arc expression in the ‘RA’ of phoebes (Spearman correlation, r =0.73; n =4). In Gambel’s quails, Arc was expressed all over the arcopallium, but there is no specialized region identified by the messenger RNA expression pattern, and no difference between silent and singing conditions ( n =3 males per group; one-way ANOVA; F =23.5; P >0.05; Fig. 2d ). 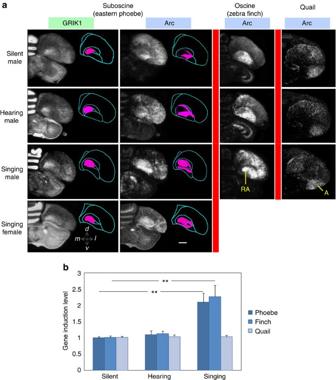Figure 2: Singing-regulated gene expression in the RA-like region of eastern phoebes. (a) Dark field images ofin situhybridization showing increased expression of the activity-regulated immediate early geneArc(right panels) in theGRIK1-rich RA-like region (adjacent sections in left panels) of singing phoebes, compared to hearing song only and silent controls (coronal view of the right hemisphere). The expression pattern in the RA-like area is highlighted in the drawings immediately right to the dark field images. (b) In oscine songbird, singing causes upregulation ofArcin zebra finch RA. (c) No specialized area of vocalizing-drivenArcexpression can be identified in the arcopallium of the Gambel’s quail. Scale bar, 1 mm. (d) Quantification ofArcexpression in the RA-like area among silent (n=3 birds), hearing (n=3) and singing (n= 4) groups (one-way ANOVA,F=5.61;P<0.001) of phoebes (suboscine), zebra finch (oscine), and Gambel’s quail (Galliformes). The gene induction values are relative to average of silent controls; induction level >1 indicates higherArcexpression than in silent birds. Error bars are s.e.m. Figure 2: Singing-regulated gene expression in the RA-like region of eastern phoebes. ( a ) Dark field images of in situ hybridization showing increased expression of the activity-regulated immediate early gene Arc (right panels) in the GRIK1 -rich RA-like region (adjacent sections in left panels) of singing phoebes, compared to hearing song only and silent controls (coronal view of the right hemisphere). The expression pattern in the RA-like area is highlighted in the drawings immediately right to the dark field images. ( b ) In oscine songbird, singing causes upregulation of Arc in zebra finch RA. ( c ) No specialized area of vocalizing-driven Arc expression can be identified in the arcopallium of the Gambel’s quail. Scale bar, 1 mm. ( d ) Quantification of Arc expression in the RA-like area among silent ( n =3 birds), hearing ( n =3) and singing ( n = 4) groups (one-way ANOVA, F =5.61; P <0.001) of phoebes (suboscine), zebra finch (oscine), and Gambel’s quail (Galliformes). The gene induction values are relative to average of silent controls; induction level >1 indicates higher Arc expression than in silent birds. Error bars are s.e.m. Full size image In contrast to Arc , singing in phoebes did not induce significantly higher expression of Egr1 in the RA-like region (one-way ANOVA, F =1.35, P >0.05; Fig. 3 ), and the expression level was significantly lower than in the surrounding arcopallium, suggesting Egr1 in the arcopallium may be associated with other motor-or sensory-related activity instead of singing. Also, singing did not induce higher Egr1 expression in the dorsal nidopallium (Nd, where the song nucleus HVC is located in oscines; singing induces Egr1 expression in HVC [34] ) compared to a hearing-only group (one-way ANOVA, F =0.98; P >0.05). Taken together, these results suggest that the GRIK1 -rich RA-like region in the suboscine phoebe is associated with singing, but lacks expression of some singing-regulated genes that are present in the songbird’s RA. 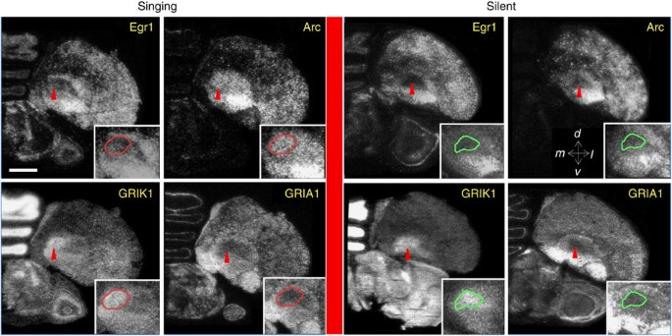Figure 3: Singing in phoebes does not induceEgr1 expression in theGRIK1-rich arcopallium region. Egr1shows significantly higher expression levels in the surrounding arcopallium region, but notGRIK1-rich, GRIA1-poor region (red arrow), during both singing, and hearing of con-specific song playback, which has been shown to be due to either hearing sounds or movement in birds generally. The insets with red and green circles outline theGRIK1-rich, GRIA1-poor RA-like area in singing and silent phoebes respectively. The insets are X1.7 higher magnification in relation to the larger panel. Scale bar, 1 mm. Figure 3: Singing in phoebes does not induce Egr 1 expression in the GRIK1 -rich arcopallium region. Egr1 shows significantly higher expression levels in the surrounding arcopallium region, but not GRIK1 -rich, GRIA1-poor region (red arrow), during both singing, and hearing of con-specific song playback, which has been shown to be due to either hearing sounds or movement in birds generally. The insets with red and green circles outline the GRIK1 -rich, GRIA1-poor RA-like area in singing and silent phoebes respectively. The insets are X1.7 higher magnification in relation to the larger panel. Scale bar, 1 mm. Full size image RA-like region connects to brainstem respiratory nucleus We further conducted tract-tracing studies to test whether the arcopallium’s RA-like area connects to the midbrain and medulla vocal-motor and respiratory nuclei in phoebes. A lipophilic carbocyanine dye, DiIC 12 , was injected into the GRIK1 -rich, RA-like region in phoebes ( Fig. 4 ). In the descending pathway, projection fibres labelled with DiI exited the RA-like region rostrally and entered the occipitomesencephalic tract, which projects from the forebrain to the thalamus, and then travelled around nucleus Ovoidalis (Ov, Fig. 4a ) of the thalamus, which is part of the ascending auditory pathway. In the midbrain, some labelled fibres left occipitomesencephalic tract and coursed laterally into the intercollicular region. While some of these fibres entered the dorsomedial (DM) nucleus of the intercollicular region, others travelled around the nucleus mesencephalicus lateralis, pars dorsalis (MLd), the avian inferior colliculus ( Fig. 4b ), which is also a part of the ascending auditory pathway. Another cohort of labelled fibres reached the medulla. Some of these fibres ended in a dense terminal field that arched laterally and ventrolaterally from the hypoglossal nucleus across the dorsal central medulla. The more medial part of this arc included relatively large cells presumed to be motor neurons that, by similarity with the zebra finch brain, were judged to correspond to nucleus ambiguous, which innervates the larynx ( Fig. 4d ). Caudal to nucleus ambiguous, the labelled fibres entered the respiratory pre-motor nucleus retroambigualis (RAm) [35] , [36] ( Fig. 4e–g ). We found no strong, direct link between the arcopallium’s RA-like region and the brainstem hypoglossal nucleus ‘nXIIts’, which innervates muscles of the trachea and syrinx. 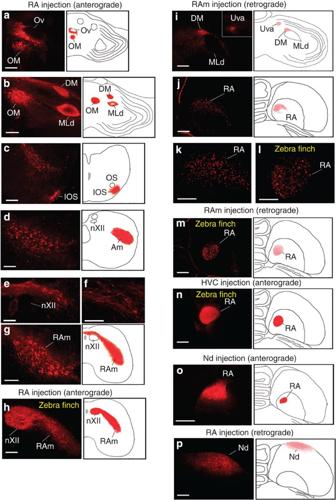Figure 4: Tract-tracing reveals connections between the forebrain and midbrain/brainstem motor-respiratory pathway in suboscine phoebes. Connectivity from injections of tracer (DiI,C12) into the intermediateGRIK1-rich, RA-like area of the pheobe arcopallium. (a) Anterogradely labelled fibre bundles travelled around Ov and through OM; many ended in the midbrain vocal-motor nucleus, DM, and surrounded the adjacent auditory region, nucleus mesencephalicus lateralis, pars dorsalis (MLd) (b). Projections further travelled down the brainstem via the IOS (nucleus infra-olivarus superior) around nucleus OS (c). These axons travelled down to nucleus ambiguous but did not innervate tracheosyringeal hypoglossal nucleus (nXII) (d,e), and further terminated in the brainstem respiratory nucleus RAm (g); with a higher magnification showing labelled fibre terminals (f). (h) Injection of DiI in song nucleus RA of a songbird, the zebra finch, anterogradely labelled nXII and RAm. Connectivity from injections of DiI tracer into the pheobe’s RAm. (i) Retrogradely labelled cells in the midbrain vocal nucleus DM but not auditory nucleus MLd, and in an Uva-like song nucleus in the thalamus. (j) Retrogradely labelled cell bodies in theGRIK1-rich, RA-like region, confirming this projection; the labelled cell bodies are also shown in a higher magnification (k); and this retrograde labelling is comparable to the DiI injection of RAm in the zebra finch (l). (m) DiI injection in RAm of a male zebra finch retrogradely labelled cell bodies of song nucleus RA in the arcopallium. (n) DiI injection in the zebra finch nucleus HVC anterogradely labeled nucleus RA. (o) Injection in Nd anterogradely labelled RA-like region in intermediate arcopallium, whereGRIK1is highly expressed, confirming this projection. (p) Injection of DiI in the pheobe’s RA-like region retrogradely labelled cells in the Nd. Scale bar, 0.5 mm. Figure 4: Tract-tracing reveals connections between the forebrain and midbrain/brainstem motor-respiratory pathway in suboscine phoebes. Connectivity from injections of tracer (DiI,C12) into the intermediate GRIK1 -rich, RA-like area of the pheobe arcopallium. ( a ) Anterogradely labelled fibre bundles travelled around Ov and through OM; many ended in the midbrain vocal-motor nucleus, DM, and surrounded the adjacent auditory region, nucleus mesencephalicus lateralis, pars dorsalis (MLd) ( b ). Projections further travelled down the brainstem via the IOS (nucleus infra-olivarus superior) around nucleus OS ( c ). These axons travelled down to nucleus ambiguous but did not innervate tracheosyringeal hypoglossal nucleus (nXII) ( d , e ), and further terminated in the brainstem respiratory nucleus RAm ( g ); with a higher magnification showing labelled fibre terminals ( f ). ( h ) Injection of DiI in song nucleus RA of a songbird, the zebra finch, anterogradely labelled nXII and RAm. Connectivity from injections of DiI tracer into the pheobe’s RAm. ( i ) Retrogradely labelled cells in the midbrain vocal nucleus DM but not auditory nucleus MLd, and in an Uva-like song nucleus in the thalamus. ( j ) Retrogradely labelled cell bodies in the GRIK1 -rich, RA-like region, confirming this projection; the labelled cell bodies are also shown in a higher magnification ( k ); and this retrograde labelling is comparable to the DiI injection of RAm in the zebra finch ( l ). ( m ) DiI injection in RAm of a male zebra finch retrogradely labelled cell bodies of song nucleus RA in the arcopallium. ( n ) DiI injection in the zebra finch nucleus HVC anterogradely labeled nucleus RA. ( o ) Injection in Nd anterogradely labelled RA-like region in intermediate arcopallium, where GRIK1 is highly expressed, confirming this projection. ( p ) Injection of DiI in the pheobe’s RA-like region retrogradely labelled cells in the Nd. Scale bar, 0.5 mm. Full size image Injections of DiI into nucleus retroambigualis, RAm, verified that it receives a projection from the RA-like region. RAm also projects to an ‘Uva-like’ (nucleus uvaeformis) area of the thalamus, and retrogradely labelled nucleus DM and the GRIK1 -rich RA-like region in the arcopallium of phoebes ( n =3 birds; Fig. 4j ). The injections of DiI into the phoebe’s RA-like region also retrogradely labelled cell bodies in the dorsal Nd where the oscine’s song nucleus HVC is located. However, unlike HVC, this region was diffuse and did not have the clear cytoarchitectonic boundaries that define the oscine HVC ( n =3 birds, Fig. 4p ). In contrast to the oscine RA’s connections from anterior Nd song nucleus, lMAN, there was diffuse labelling in the more medial part of anterior Nd in phoebes (data not shown). Injections of DiI into Nd verified labelled fibre projections that ended in the RA-like region ( Fig. 4o ). However, we could not find a recognizable anterior projection from Nd to the anterior striatum (where song nucleus Area X is located), an important projection in the song system of oscines. These results suggest that phoebes have a descending motor pathway from a specialized subregion of the arcopallium that is reminiscent of nucleus RA in oscines and that this pathway is active during song production. However, we have no evidence that phoebes have an anterior loop that in oscines connects HVC to Area X and that receives input from lMAN to RA. This anterior forebrain loop identified in oscines has an important role for vocal learning. Bilateral lesion of RA-like region induces vocal changes To further assess the function of the specialized RA-like region in phoebes, adult male phoebes received bilateral lesions in the GRIK1 -rich RA-like region ( n =4, two of them received nearly complete lesions). The adult phoebe song has two alternating song types ( Fig. 5 ). Three weeks after surgery, the two song types of postoperative birds showed subtle but significant vocal changes from preoperative renditions (multivariate analysis of variance (MANOVA), Wilks’ lambda=0.59, F =43.7, P <0.01, Fig. 5 ). Acoustic features, such as frequency modulation, Wiener entropy, duration and pitch, became more variable and showed significant changes in post-lesion birds, but the effect varied individually ( Fig. 6 ; Supplementary Table S1 ). No systematic vocal differences were identified in control birds that received bilateral lesion near the RA-like region (MANOVA, F =26.5, P >0.05; n =3 birds). In addition, bilateral lesions of Nd (where oscine’s nucleus HVC is located) in phoebes produced no significant difference in song features after surgery ( n =3 birds, MANOVA, Wilks’ lambda=0.24; F =31.3, P >0.05). 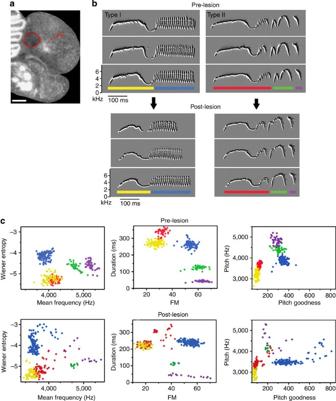Figure 5: Electrolytic lesion of theGRIK1-rich RA-like region induces acoustic changes of phoebe song. (a) Coronal view of lesion site, highlighted in the red circle. The postoperative phoebe was later used forin situhybridization of parvalbumin to demonstrate that the lateral part of arcopallium remains intact. Scale bar, 1 mm. (b) Three example sonograms of the two song types (Type I and II) produced by an adult male before and after electrolytic lesions. Below the sonograms are coloured bars that denote single song notes of each of the songs. Note the change in reduced stereotypy after the lesion. All of the songs were recorded in the late morning (0800–1200) during the breeding season; (c) cluster analysis of six sound features (seeMethodsfor details) for each of five notes from the two song types of the same individual in panel (b). Colours match the notes shown in panel (b), before and after surgery. This analysis was conducted by automated categorization and clustering of the song notes, defined by continuous sound produced at note–note interval of less than 10 ms. The mean frequency, FM, pitch and duration of the syllables changed significantly after lesion with greater variability in these acoustic features. Figure 5: Electrolytic lesion of the GRIK1 -rich RA-like region induces acoustic changes of phoebe song. ( a ) Coronal view of lesion site, highlighted in the red circle. The postoperative phoebe was later used for in situ hybridization of parvalbumin to demonstrate that the lateral part of arcopallium remains intact. Scale bar, 1 mm. ( b ) Three example sonograms of the two song types (Type I and II) produced by an adult male before and after electrolytic lesions. Below the sonograms are coloured bars that denote single song notes of each of the songs. Note the change in reduced stereotypy after the lesion. All of the songs were recorded in the late morning (0800–1200) during the breeding season; ( c ) cluster analysis of six sound features (see Methods for details) for each of five notes from the two song types of the same individual in panel ( b ). Colours match the notes shown in panel ( b ), before and after surgery. This analysis was conducted by automated categorization and clustering of the song notes, defined by continuous sound produced at note–note interval of less than 10 ms. The mean frequency, FM, pitch and duration of the syllables changed significantly after lesion with greater variability in these acoustic features. 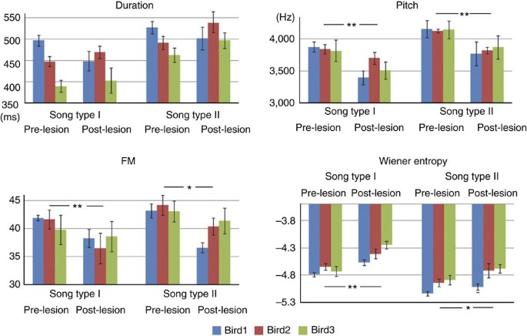Figure 6: Effects of bilateral ‘RA’ lesions on key features of phoebe song. Here we illustrate significant change in four song features (song duration, pitch, frequency modulation, FM and Wiener entropy) in two song types (I and II), before and after ‘RA’ lesions. ANOVA was used to test the overall significant change in each of the acoustic features in three experimental birds. The fourth bird was not included because it did not sing the second song type (song type II) after lesioning. The first two birds received complete bilateral lesions of ‘RA’, the third and fourth birds received complete lesion only unilaterally, but partial lesion in the other hemisphere. Asterisk (*) denotes a change significant atP<0.05; double asterisk (**) denotes a change significant atP<0.01. Error bars are s.e.m. Full size image Figure 6: Effects of bilateral ‘RA’ lesions on key features of phoebe song. Here we illustrate significant change in four song features (song duration, pitch, frequency modulation, FM and Wiener entropy) in two song types (I and II), before and after ‘RA’ lesions. ANOVA was used to test the overall significant change in each of the acoustic features in three experimental birds. The fourth bird was not included because it did not sing the second song type (song type II) after lesioning. The first two birds received complete bilateral lesions of ‘RA’, the third and fourth birds received complete lesion only unilaterally, but partial lesion in the other hemisphere. Asterisk (*) denotes a change significant at P <0.05; double asterisk (**) denotes a change significant at P <0.01. Error bars are s.e.m. Full size image Protracted song ontogeny in juvenile phoebes Lastly, we tested whether the unlearned song produced by adult phoebes requires a protracted ontogeny that has been characterized in oscines. In oscines, the development of learned vocalizations starts with soft and highly variable babbling sounds (that is, subsong), as juveniles gradually modify their vocal output by reference to an external model. We expected that the unlearned song of phoebes would first arise already well developed and with limited variability, as seen in another avian non-vocal-learner, quails [37] . As predicted, the early ‘prototypes’ of the phoebe’s two song types emerged as early as 1–2 months after hatching, but these plastic songs remained highly variable and continued to slowly change in song features for the next 7–8 months ( Fig. 7 ). As the breeding season approached, the amount of plastic song surged and was accompanied with intense wing flapping ( Supplementary Movie 1 ). The song then became crystallized in a few weeks, as the Wiener entropy was significantly reduced and pitch increased ( Fig. 7 ). This prolonged period of singing and surge in plastic song production before crystallization is similar to that seen in an oscine, the chipping sparrow ( Spizella passerina , Fig. 7e ). 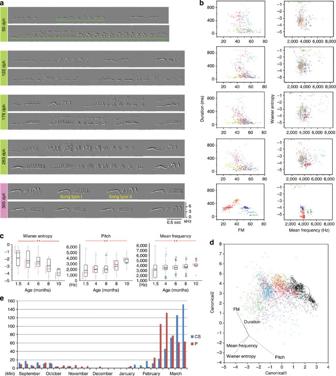Figure 7: Development of phoebe song. (a) An example of the song ontogeny in the eastern phoebe. This bird was raised without exposure of con-specific adults. An approximation of the adult form of phoebe song was already produced by 50 days post hatching (d.p.h.), this ‘prototype’ song was highly variable and was intermingled with a long series of soft vocalizations (underlined in green) in each singing bout. Both vocalizations were gradually modified with age and became crystallized by the breeding age, at approximately 10 months of age. Below the sonograms of crystallized song are coloured dots that denote single song notes shown in (b). (b) Corresponding to each age stage of song ontogeny shown in (a), we used cluster analysis to show the highly variable songs produced as juveniles and were slowly but gradually changed in some of the acoustic features, and eventually crystallized as adults (~305 dph). Each colour dot represents a sound note (defined by a time interval of 10-ms silence between two notes) produced by phoebes and categorized by cluster analysis using six sound parameters (seemethodsfor details). (c) developmental changes of the song features. Three acoustic features of the song: Wiener entropy, pitch and mean frequency show significant developmental differences over the first 10 months of age (one-way ANOVA, **=P<0.01;n=4 birds, mean (diamond shape) and median (line) are shown in each box plot). (d) Discriminant function analysis, using a combination of five song features, shows the significant differences between juvenile plastic song (coloured dots) at age of 6 month old and adult crystallized song (black dots) crystallized at 10 month old (n=3 birds). (e) The amount of singing (recorded once a week) produced throughout the first year of seasonal phoebes;P=the eastern phoebe;n=3 birds); CS=the chipping sparrow, a seasonal songbird for comparison (n=5). Both species significantly increased the amount of singing during the early spring, when chipping sparrows produced the ‘plastic song’ and phoebes produced intense vocalizations and songs. As with oscine songbirds, when phoebe songs became crystallized in March, the amount of singing was significantly reduced. Figure 7: Development of phoebe song. ( a ) An example of the song ontogeny in the eastern phoebe. This bird was raised without exposure of con-specific adults. An approximation of the adult form of phoebe song was already produced by 50 days post hatching (d.p.h. ), this ‘prototype’ song was highly variable and was intermingled with a long series of soft vocalizations (underlined in green) in each singing bout. Both vocalizations were gradually modified with age and became crystallized by the breeding age, at approximately 10 months of age. Below the sonograms of crystallized song are coloured dots that denote single song notes shown in ( b ). ( b ) Corresponding to each age stage of song ontogeny shown in ( a ), we used cluster analysis to show the highly variable songs produced as juveniles and were slowly but gradually changed in some of the acoustic features, and eventually crystallized as adults (~305 dph). Each colour dot represents a sound note (defined by a time interval of 10-ms silence between two notes) produced by phoebes and categorized by cluster analysis using six sound parameters (see methods for details). ( c ) developmental changes of the song features. Three acoustic features of the song: Wiener entropy, pitch and mean frequency show significant developmental differences over the first 10 months of age (one-way ANOVA, **= P <0.01; n =4 birds, mean (diamond shape) and median (line) are shown in each box plot). ( d ) Discriminant function analysis, using a combination of five song features, shows the significant differences between juvenile plastic song (coloured dots) at age of 6 month old and adult crystallized song (black dots) crystallized at 10 month old ( n =3 birds). ( e ) The amount of singing (recorded once a week) produced throughout the first year of seasonal phoebes; P =the eastern phoebe; n =3 birds); CS=the chipping sparrow, a seasonal songbird for comparison ( n =5). Both species significantly increased the amount of singing during the early spring, when chipping sparrows produced the ‘plastic song’ and phoebes produced intense vocalizations and songs. As with oscine songbirds, when phoebe songs became crystallized in March, the amount of singing was significantly reduced. Full size image The prolonged 8–9 months of phoebe’s plastic song singing always included a long series of vocalizations ( Fig. 7a ). These diverse vocalizations were predominantly produced as part of singing bouts and seem inseparable from the song, as they were intermingled with each other, both are acoustically similar, and both were simultaneously and progressively changed in acoustic features with age ( Fig. 7a ). When song crystallized, phoebes stopped singing these vocalizations and wing flapping diminished ( Supplementary Movie 1 ). The crystallized, long series of vocalizations are reminiscent of the adult ‘chatter calls’ produced during the flight-song display [38] . Our study provides the first evidence that non-vocal-learning phoebes possess some of the forebrain vocal/respiratory control that are required for vocal learning in oscines, though their exact role in phoebes is not clear. The rudimentary circuitry had not been observed in other avian non-vocal-learners ( Fig. 8 ). In oscines, song nucleus RA is the main output of the forebrain song system, and descending projections from RA terminate directly on the brainstem respiratory and vocal-motor neurons. We suggest that the ‘ GRIK1 -rich’ region in the Ai of phoebes is homologous to the oscine RA nucleus because of its connectivity, gene expression pattern and singing-associated function. A similar RA-like region in arcopallium can also be identified by GRIK1 and GRIA1 in two other tyranni suboscines (Liu, unpublished data). However, the phoebe’s RA-like region is different from that of oscines because of the lack of expression of certain genes (that is, GRM2, GRIN2A, PV , Egr1, and dusp1 (ref. 19 )) that are found expressed in the oscine RA; because there is no direct projection from it to the tracheosyringeal hypoglossal nucleus; and the lack of connections to the other forebrain regions that are important for vocal learning. 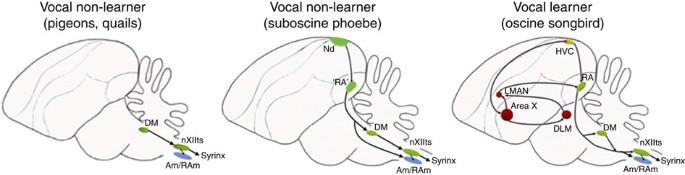Figure 8: A tentative and schematic representation of vocal control pathways in suboscine phoebes. Vocal learning oscines are characterized by a specialized forebrain song system that is essential for vocal learning and production of learned sounds. It is thought that non-vocal learning avian species lack such forebrain vocal circuitry, and the midbrain/ brainstem vocal/respiratory pathway is sufficient to produce unlearned sounds. Our current study of suboscine phoebes, however, provides the first evidence of forebrain vocal-motor control in a non-vocal learning species. However, this forebrain vocal-motor pathway is rudimentary compared to the song system in songbirds, due to its lack of connection to the anterior forebrain basal ganglia circuit and functionally different RA-like area. This rudimentary pathway bridges an important missing evolutionary gap in the study of vocal learning in songbirds. Figure 8: A tentative and schematic representation of vocal control pathways in suboscine phoebes. Vocal learning oscines are characterized by a specialized forebrain song system that is essential for vocal learning and production of learned sounds. It is thought that non-vocal learning avian species lack such forebrain vocal circuitry, and the midbrain/ brainstem vocal/respiratory pathway is sufficient to produce unlearned sounds. Our current study of suboscine phoebes, however, provides the first evidence of forebrain vocal-motor control in a non-vocal learning species. However, this forebrain vocal-motor pathway is rudimentary compared to the song system in songbirds, due to its lack of connection to the anterior forebrain basal ganglia circuit and functionally different RA-like area. This rudimentary pathway bridges an important missing evolutionary gap in the study of vocal learning in songbirds. Full size image Our results may shed light on the evolution of vocal-learning circuits, which have been proposed to have emerged either from a descending auditory pathway that then added a motor function [39] , [40] ; or, conversely, that motor pathways became overlaid by auditory control [41] . It has been suggested that in pigeons (Columbiformes), part of the Nd and Ai are thought to be homologous to the auditory ‘shelf’ and the auditory ‘cup’ adjacent to the oscine HVC and RA respectively. Like phoebe’s Nd and the RA-like region, the HVC shelf projects to the RA cup, and the RA cup to the shell auditory regions around Ov and MLd. Because of the immediate proximity in oscines between the auditory relays and song nuclei, and the fact that pre-motor neurons in HVC and RA can also be driven by sound, it is tempting to speculate that forebrain control and the vocal learning function of the oscine song system evolved from circuits initially used for auditory processing. However, the RA cup in oscines and the Ai of pigeons do not project to vocal and respiratory nuclei of the midbrain, (DM) and medulla (RAm), nor does it play a role in vocalization [42] . The exact relation between forebrain control of vocalization and auditory relays has been described in much less detail in parrots [9] , [43] . Furthermore, the wing flapping behaviour associated with phoebe plastic song suggests a potential link between song production and a complementary motor behaviour in phoebes. Because the occipitomesencephalic tract that carries the output from RA also carries other motor output from the arcopallium, there is this anatomical proximity between song and other motor activity that occurs at the same time as birds sing [41] . In phoebes, the RA-like region seems to have characteristics of both the descending vocal-motor and auditory pathways, whereas in songbirds they are more separate. This RA-like region projects around the descending auditory pathway of the Ov and MLd, but then also projects to midbrain and brainstem vocal/respiratory nuclei presumably involved in vocal control. This blending of seemingly auditory and vocal function in the RA-like region of phoebes could be close to one of the preconditions necessary for the emergence of vocal learning and provides an important evolutionary bridge between non-vocal-learners and vocal learners. Song ontogeny in phoebes presents similarities to song development of another non-vocal-learner, the Japanese quail ( Coturnix coturnix japonica ), as both show vocal variability and developmental changes in song structures [37] . The song variability in both species might be associated with the seasonal changes in hormone levels [44] , developmental changes in vocal/ respiratory circuits, or anatomical maturation in vocal organ and peripheral vocal apparatus [45] , [46] , [47] . Unlike quails, however, juvenile phoebes have a protracted 8–9 months of song ontogeny, which incorporates a much greater diversity of sounds. This phoebe song development is more closely reminiscent of the song ontogeny of oscines than that of quails. Young seasonal songbirds produce subsong or plastic song during a prolonged period before they reach sexual maturity [48] ( Fig.7 ). During this period, songbirds often ‘overproduced’ plastic songs [48] . In chipping sparrows, for example, juveniles produce several different song prototypes before the breeding season begins. One of these prototypes is selectively modified to match a tutor song and then crystallized. Some of these sounds may be used as acoustic reference to fine-tune the acoustic features of the song they produced [39] . And these sounds cease to be used after crystallization. The function of diverse sounds predominantly produced during the song ontogeny of phoebes remains to be tested. The unexpected length of song ontogeny suggests that substantial practice of vocal and respiratory control is required for phoebe’s song development. However, because phoebes do not learn their song under auditory guidance [18] , what might be the purpose of the juvenile singing? This ontogeny might help phoebes to more precisely control their song with expiration, or to fine tune some of the song features. Adult phoebes have a spectacular aerial ‘flight-song’ display during the early breeding season. This aerial song display, which includes continuous singing while hovering high in the air (Liu, personal observations [38] ), may require substantial vocal/respiratory coordination and practice, as the oscine songbird has to learn to breathe and sing during song development [49] . This elaborate aerial song display may provide an honest signal for inter- or intrasexual selection, similar to the aerial vocal display of hummingbirds or Alauda skylarks [50] , [51] . And we predict a specialized forebrain pathway for finer vocal/respiratory control may enable aerial song display that is also commonly seen in suboscine flycatchers (tyrannidae) [52] or manakins (pipridae) [24] . The effect of ‘RA’ lesions on phoebe song is similar to the effect of RA lesion on zebra finches’ learned calls [8] , [53] . In zebra finches, only males sing and their song and ‘long call’ are learned. Bilateral lesion of the zebra finch’s RA completely abolishes song production [47] , but their learned calls persist. However, following RA lesion the duration and frequency modulation of the learned calls become more variable. This observation suggests that despite difference in connectivity and cytochemistry, the RA of zebra finches and the RA-like region of phoebes share a partial functional similarity in vocal control. It remains to be tested whether the RA-like region of phoebes influences the duration of expiration during singing, and so affects the length of song duration and fine control of song stereotypy. Recent studies of avian phylogeny show two vocal-learning clades, parrots and songbirds, now reclassified as close sister groups ( Fig.1a ) [54] , [55] . Perhaps vocal learning was already present in the ancestor of both Psittaciformes and Passeriformes, and the suboscines secondarily lost their potential for vocal learning. The neural and behavioural substrates we described in phoebes may thus represent the vestige of complex vocal-learning circuitry. Alternatively, the forebrain pathways for respiratory control of vocalizations observed in phoebes might have been common to the ancestor of Passeriformes and Psittaciformes and then separately enabled and given rise to vocal learning in oscines and parrots (that is, parallel evolution) [17] . Another avian vocal-learning group, the hummingbird (Apodiformes), is thought to have evolved vocal learning independently from the ancestors of parrots and oscines. All of these vocal learners share relatively small body size [56] , which may allow these birds (and their ancestors) to better manoeuvre flight and create more ecological niches [56] for foraging (nectar feeding, flying-insect catching) and aerial vocal display. Such elaborate flight manoeuvreing may require a better coordination or reconfiguration of respiratory control from the forebrain. The forebrain respiratory control may subsequently integrate pre-existing motor pathway in the arcopallium for the control of flight, jaw, and vocal movement [11] , [41] , and/or auditory relays [57] , and lead to evolution of vocal learning (see a similar view proposed by Janik and Slater [58] for vocal learning in mammals). Although this ‘respiratory control’ hypothesis is highly speculative, the diversity of vocal plasticity, syringeal structure, and neural substrate observed among suboscine species suggest further study of suboscines may help unravel the behavioural, genetic, and anatomical origin of vocal learning. Experimental subjects A suboscine passerine, the eastern phoebe, was chosen as the experimental subject. Eastern phoebes are a seasonal migratory birds of the northeastern America. There were practical limitations on collecting limited number of wild phoebes and hand rear them in the present study. Nestling phoebes ( n =33 birds) were collected at post-hatching days 7–11 from nests at the Rockefeller University Field Research Center in Millbrook, New York. Juveniles were hand reared until independence (at post-hatching days 35–40). Due to the limitations on the number of birds collected in the wild, some of these birds were repeatedly used for two or more experiments. The sex of each individual bird was first determined from blood samples using polymerase chain reaction amplification of CHD gene fragments following the protocol of Griffiths et al . [59] We also used Gambel’s quails ( n =7 adult males) for a comparative study of gene expression. The quails were purchased from a local farm, and the sex was determined by the plumage and vocalization and later confirmed by gonadal examination. Two songbird species, the chipping sparrow ( Spizella passerina ; n =3) and zebra finch ( Taeniopygia guttata ; n =3), were also used in this study. These animals and their brain sections had been collected during a previous study [38] . Animal procedures were reviewed and approved as meeting appropriate ethical standards by The Rockefeller University's IACUC board. In situ hybridization For in situ hybridization of activity-dependent immediate early gene expression, we collected brains from three groups of adult animals: silent controls ( n =4), hearing ( n =3), and singing ( n = 3). After sexual maturity (260–280 dph) in the spring, each bird was individually housed in a sound isolation chamber, and was killed in the morning approximately 45 min after lights were turned on. The birds were killed either (1) after 45 min of silence; (2) after 30 min of hearing of con-specific song playback with 7–10 songs per minute (both song types), followed by 15 min of silence; or (3) singing for at least 15 min (or >100 songs) and killed 45 min after singing began. The birds in the hearing-only group occasionally produced contact calls during the 45-min period. Adult phoebe vocalizations were recorded with Raven 1.2 software (Cornell laboratory of Ornithology, Ithaca, New York). We counted the number of songs produced by each bird by examining the spectrograms from our continuous recordings. For Gambel’s quails, birds were assigned to three experimental groups: silent controls ( n =3 males), hearing ( n =3 males), and singing group ( n =4 males): In the singing group, birds were singing song alone for 15–45 min, they were killed 1 h after started singing. The experimental and recording conditions were similar to that used for phoebes. The animals were kept in an isolation room overnight, and brains were collected for groups depending on the planned conditions and their behavior. After sacrificing the birds, their brains were removed and embedded in OCT compound (Sakura Fine Technical, Tokyo, Japan), frozen and stored at −80 o C. In situ hybridizations were performed and quantified following a protocol described previously [60] using 33 P-labelled riboprobes. In brief, frozen brain sections (14 μm) were hybridized with 33 P-labelled antisense riboprobes of zebra finch GRIA1, GRIK1, GRM2, GRIN2A , Egr1 and Arc , as described in previous studies [28] , [33] , [34] . The sections were overlaid by x-ray film for 1–5 days. After developing the X-ray films (Biomax MR, Kodak, Rochester, NY), then dipped into autoradiographic emulsion (NTB2, Kodak), incubated for 3 weeks, processed with D-19 developer (Kodak) and fixer (Kodak), Nissl-stained with 3% cresyl -violet acetate solution (Sigma, St. Louis, MO), and coverslipped. Quantification and statistics Gene expression level in the specialized arcopallium region was quantified following a previously described procedure with modifications. In brief, the brain image on the exposed film was placed and scanned under a photo scanner scanned with 5000, d.p.i. (Epson, Perfection V700, Long Beach, CA). Images were then exported to Adobe Photoshop CS2 (Adobe, San Jose, CA) and converted to a 256 grey scale. The glutamate receptor-rich RA-like region and surrounding arcopallium areas were outlined and the average pixel density was calculated using the Photoshop histogram function. To quantify and compare the relative amount of Arc or egr1 expression in the RA-like nuclei of the singing or hearing animals relative to non-singing silent controls, we normalized the amount of Arc or egr1 expression in each song nucleus by the average amount in silent controls. Statistical differences were determined by one-way ANOVA for overall differences between silent controls and singing groups for each gene we tested. To examine the amount of singing as a variable, we performed a regression analysis on total time spent singing (in seconds) for each animal of the 45-min singing group versus the amount of IEG ( Arc and Egr1 ) expression in each nucleus. Tract-tracing We used tract tracers, carbocyanines dye, DiIC 12 , injecting into ( A) the GRIK1 -rich, RA-like area in the arcopallium of phoebes; ( B) dorsal Nd in the midbrain; and ( C) retroambigulias (RAm) in the brainstem. Anaesthesia was first induced with intramuscular injection of Nembutal (1:5) and maintained by 1–1.5% isofluorane. The scalp was then retracted and a small craniotomy made over the injection site. Injections of DiI were made through a glass micropipette using the Nanoject II microinjector (Drummond Scientific). For each nucleus, four 50–100 nL injections were made with 45 s apart. The birds were then killed 1–2 weeks after injection and the brain was sectioned with cryostat at 20 μm. Injection sites and track-tracing areas were examined with microscopy. Electrolytic lesion Adult phoebes received bilateral lesions of the RA-like specialized area ( n =4 birds) and dorsal Nd. We used size 000 insect pins (Fine Science Tools, Foster City, CA) insulated with Insl-x (Insl-X Product) as electrodes. The coordinates for Ai and dorsal Nd were obtained by trial and error with three adult phoebes, and reference to the canary brain atlas as both have similar body size. Two penetrations were made into the RA-like area and current of 50 μA for 40 s was delivered (each penetration injected at two depth) and found sufficient. For the lesion-control group ( n =3 birds), the lesion was done by two penetrations in the arcopallium outside and adjacent to the RA-like region. Each of the preoperative birds was placed in a sound-proof chamber and their vocalizations (songs and calls) were recorded for at least 3 consecutive days (recorded from 0800–1200) immediately prior to surgery. After 1 week of recovery from surgery, the postoperative birds were placed back in the sound-proof chamber. The phoebe sounds were recorded continuously for 2–3 weeks (between 0800 and 1200), approximately 200 s of sounds per bird were collected for sound analysis. To identify the effectiveness of lesions targeted at the RA-like region, postoperative birds were decapitated, and their brains were removed and sectioned (14μm) in a cryostat. Sections were stained with a 0.13% solution of cresyl violet acetate (Sigma) and tested with in situ hybridization of GRIK1 or PV to identify whether the RA-like region was lesioned. Recording of song ontogeny and sound analysis At approximate 1 month of age, juvenile phoebes were housed singly in a sound-proof chamber, with continuous recording for 6 h after lights on (note: phoebes are seasonal birds, and therefore the light cycle was adjusted according to the photoperiod in their natural habitat). For sound recordings, we used an Audio technica AT803 microphone (Audio-Technica, Stow, Ohio) connected to M-audio Audio-Buddy pre-amp (Avid Technology, Irwindale, CA), which relayed audio to a recording software designed by Tim Gardner at Boston University; phoebe vocalizations were continuously recorded for once a week from August to the next April. Sound analysis Quantitative sound analysis was performed using Sound Analysis Pro software (SAP, version 2). Each bird’s vocalizations were analysed at the level of a single note (a call note was defined as a continuous sound preceded and followed by silent intervals of >10 ms). Quantification of vocalizations was done using a similarity score obtained from asymmetric pairwise comparisons. The frequency range was adjusted to 11800 Hz in the setting of SAP. The sound intervals (9.27 ms) used for such comparisons was calculated with reference to six acoustic features: duration, pitch, frequency modulation, Wiener entropy, mean frequency and pitch goodness. SAP calculates the Euclidean distance between all interval pairs from two groups of sounds. To determine whether or not the song was different under different experimental conditions, we analysed each bird’s vocalizations at several developmental ages (see Fig. 5 ). Each bird’s vocalizations were compared using the six call parameters listed above and MANOVA and discriminant function analysis (SPSS 16.0), were used to determine whether the variability of sound features between the calls from two groups of birds of different age were significantly different from each other. We had also used MANOVA (SPSS 16.0) to determine whether there is a significant difference of sound features of the phoebe song before and after experimental lesion. Wilk’s lambda and overall F value was used to test for significance, with a Tukey’s post hoc test for each variable. How to cite this article: Liu W.-c. L. et al . Rudimentary substrates for vocal learning in a suboscine. Nat. Commun. 4:2082 doi: 10.1038/ncomms3082 (2013).